Phytochrome RNAi enhances major fibre quality and agronomic traits of the cottonGossypium hirsutumL Simultaneous improvement of fibre quality, early-flowering, early-maturity and productivity in Upland cotton ( G. hirsutum ) is a challenging task for conventional breeding. The influence of red/far-red light ratio on the fibre length prompted us to examine the phenotypic effects of RNA interference (RNAi) of the cotton PHYA1 gene. Here we show a suppression of up to ~70% for the PHYA1 transcript, and compensatory overexpression of up to ~20-fold in the remaining phytochromes in somatically regenerated PHYA1 RNAi cotton plants. Two independent transformants of three generations exhibited vigorous root and vegetative growth, early-flowering, significantly improved upper half mean fibre length and an improvement in other major fibre characteristics. Small decreases in lint traits were observed but seed cotton yield was increased an average 10–17% compared with controls. RNAi-associated phenotypes were heritable and transferable via sexual hybridization. These results should aid in the development of early-maturing and productive Upland cultivars with superior fibre quality. Light is one of the most important environmental factors controlling plant development and physiology. It affects virtually all aspects of plant growth, from seed germination to vegetative morphology, floral initiation, control of circadian rhythms, regulation of gene expression, gravitropism and phototropism [1] , [2] , [3] . Plants respond to light through several photoreceptor systems. The phytochrome red (R)/far-red (FR) photoreceptor gene family is best characterized in the model plant Arabidopsis thaliana , which has five phytochrome apoprotein genes, designated PHYA , PHYB , PHYC , PHYD and PHYE [1] . In cultivated cottons, the phytochrome gene family has particular importance because there is evidence that the FR/R photon ratio influences the length and diameter of developing fibre. For example, fibres from bolls that received a high FR/R photon ratio during development were longer than those that received normal photosynthetic light [4] . Genetic improvement of fibre quality and yield is a primary objective of cotton-breeding programmes worldwide [5] , [6] . To make cotton cultivation sustainable and competitive on the world market, it is imperative to develop early maturing, productive cotton cultivars producing finer (moderately lower micronaire (MIC)) and longer fibres with improved strength [6] . Conventional breeders have faced serious challenges because of negative correlations between fibre quality traits and yield components [6] , [7] , and between fibre quality and maturity [8] . We hypothesized that phytochrome genes could play a significant role in the regulation of cotton fibre length [9] . For this reason, we characterized the phytochrome gene family and its evolution in the A and D diploid Gossypium spp., as well as AD allotetrapoloid cottons Gossypium hirsutum and Gossypium barbadense [9] , [10] . The AD tetraploid Gossypium spp. inherited homologues of each of the canonical phytochrome apoprotein subfamilies PHYA , PHYB , PHYC and PHYE from each of the A- and D-genome diploid ancestral species. Further, both diploid and tetraploid cotton species have two divergent PHYA subfamilies, designated PHYA1 and PHYA2 , resulting from a Malvaceae-specific duplication that occurred ~14 million years ago, before the divergence of the A- and D-genome diploid genome groups of Gossypium [10] . The distribution of gene function between the two PHYA paralogues is unknown; however, previous efforts directed towards quantitative trait loci (QTL) mapping of fibre quality traits in a bi-parental population found a significant association of the PHYA1 gene with fibre length [9] . In this study, the fibre quality QTL-associated PHYA1 gene fragment was used to create a specific RNAi construct [11] to explore the biological roles of PHYA1 and (indirectly) other phytochrome genes in cotton. We somatically transformed the RNAi construct into the highly embryogenic but non-commercial Coker-312 variety, which is considered the genetic standard for cotton regeneration work [12] . When compared with control plants, we observed heritable improvement of major fibre quality traits, early-flowering, early-maturity, vigorous root and shoot development, and productivity traits through several generations of two independently derived RNAi cotton transformants. We further demonstrate that the RNAi-associated traits were transferable from somatically regenerated RNAi Coker-312 lines to other commercial Upland cultivars via conventional sexual hybridization. Our results provide the first molecular evidence of the importance of phytochromes in cotton fibre development, and show the usefulness of phytochrome-specific RNAi in simultaneously improving several important agronomic and fibre quality traits—a goal that has proven difficult to achieve via conventional breeding [6] . These results open a new avenue for cotton breeders to rapidly develop early-maturing and productive elite Upland cultivars with superior fibre qualities. Transformation and phenotypic evaluation in T 0 –T 3 We successfully obtained transgenic plant embryos bearing the cotton PHYA1 RNAi construct ( Fig. 1a ) that were resistant to kanamycin, the selectable marker. Compared with 15 somatically regenerated non-transformed controls, all 68 candidate PHYA1 RNAi cotton plants showed comparatively rapid and vigorous lateral and main root development and elongated petioles ( Fig. 1b ; Supplementary Figs 1 and 2 ). Fibres obtained from transgenic T 0 RNAi plants were at least 5 mm (17%) longer than fibres on control plants that were somatically regenerated using the same media and conditions ( Fig. 1c ). PCR analysis confirmed the presence of the RNAi construct in genomic DNAs of T 0 and T 1 plants ( Supplementary Fig. 3 ), and the stable Mendelian inheritance of the transgene in subsequent generations. Compared with the control genotypes lacking the RNA construct (non-transformed Coker-312 and null segregant progeny from transformed T 1 lines), the RNAi-positive families had more vigorous vegetative growth ( Figs 2a–e and 3a ) and 5–10 days earlier flowering and earlier boll maturing phenotypes ( Fig. 2a–c ; Supplementary Fig. 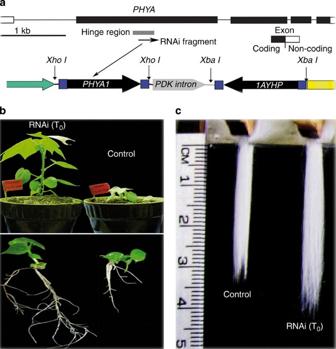Figure 1: Effects ofPHYA1RNAi in cotton. (a) Schematic representation ofPHYAgene, RNAi fragment position and pHellsgate-8::PHYA1RNAi plasmid; (b) shoot and root development and (c) fibre length characteristics of T0-generationPHYA1RNAi and control cotton plants, somatically regenerated by tissue culture. PDK intron—a pyruvate dehydrogenase kinase intron; blue boxes representattsites attached to the target gene fragment. 4 ), significantly (analysis of variance (ANOVA), P ≤0.01) longer hypocotyls ( Supplementary Figs 5 and 6 ; Supplementary Table 1 ), higher root mass and higher germination rate ( Fig. 4 ; Supplementary Fig. 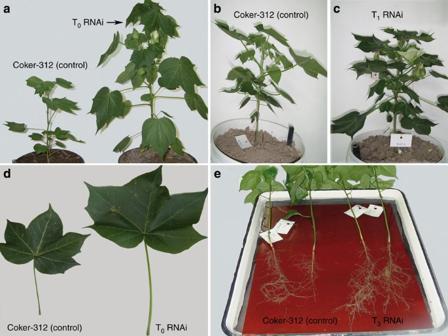Figure 2: Phytochrome-associated developmental changes inPHYA1RNAi plants. (a) Enhanced vegetative growth and early flowering in T0RNAi plants; early flowering in T1generation RNAi plant (b,c); (d) difference in petiole length (T0); and (e) difference in root development (T3). 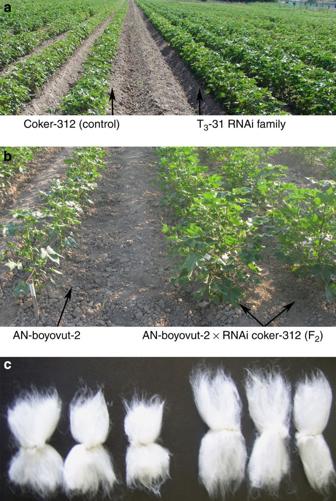Figure 3: Differences in vegetative growth between field-grown T3RNAi and control plants. Transferability of the phytochrome-associated RNAi effects from RNAi Coker-312 to Upland cultivar (AN-Boyovut-2) is shown. Enhanced plant development in the field test during 2009 (a,b); and improvement of fibre samples (c) in the original cultivar (left) and RNAi F2hybrids (right) grown in the same environment. 5 ; Supplementary Table 1 ), and more flowers and bolls ( Supplementary Table 2 ) that opened earlier ( Supplementary Table 3 ) at the time of phenotypic evaluation. We also observed elongated petioles ( Fig. 2d ), elongated boll peduncles and fruiting branches, and early senescence-associated anthocyanin pigmentation in leaves and stems ( Supplementary Fig. 4 ) in both RNAi lines. Further, when compared with near-isogenic control plants, we observed a 5–8-mm increase in fibre staple length in both PHYA1 RNAi lines ( Figs 4a and 5 ). In subsequent generations, staple length was further evaluated using high volume instrumentation. Figure 1: Effects of PHYA1 RNAi in cotton. ( a ) Schematic representation of PHYA gene, RNAi fragment position and pHellsgate-8:: PHYA1 RNAi plasmid; ( b ) shoot and root development and ( c ) fibre length characteristics of T 0 -generation PHYA1 RNAi and control cotton plants, somatically regenerated by tissue culture. PDK intron—a pyruvate dehydrogenase kinase intron; blue boxes represent att sites attached to the target gene fragment. Full size image Figure 2: Phytochrome-associated developmental changes in PHYA1 RNAi plants. ( a ) Enhanced vegetative growth and early flowering in T 0 RNAi plants; early flowering in T 1 generation RNAi plant ( b , c ); ( d ) difference in petiole length (T 0 ); and ( e ) difference in root development (T 3 ). Full size image Figure 3: Differences in vegetative growth between field-grown T 3 RNAi and control plants. Transferability of the phytochrome-associated RNAi effects from RNAi Coker-312 to Upland cultivar (AN-Boyovut-2) is shown. Enhanced plant development in the field test during 2009 ( a , b ); and improvement of fibre samples ( c ) in the original cultivar (left) and RNAi F 2 hybrids (right) grown in the same environment. 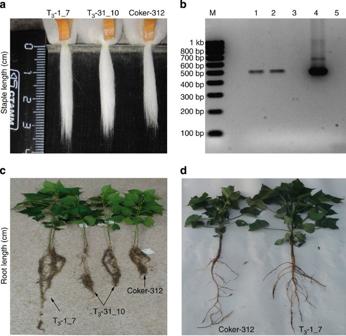Figure 4: Fibre length and root development characteristics of selected T3-generationPHYA1RNAi plant families. (a) Staple length of fibre; (b) PCR verification using 35S-F/PDK-R primer pairs (Supplementary Table 6): M-100 bp ladder, 1—T3-1_7; 2—T3-31_10; 3—Coker-312; 4—pHellsgate-8::PHYA1plasmid; 5—no DNA template control. The same plants were used for copy-number identification and relative expression analyses using qRT–PCR. Full size image Figure 4: Fibre length and root development characteristics of selected T 3 -generation PHYA1 RNAi plant families. ( a ) Staple length of fibre; ( b ) PCR verification using 35S-F/PDK-R primer pairs ( Supplementary Table 6 ): M-100 bp ladder, 1—T 3 -1_7; 2—T 3 -31_10; 3—Coker-312; 4—pHellsgate-8:: PHYA1 plasmid; 5—no DNA template control. 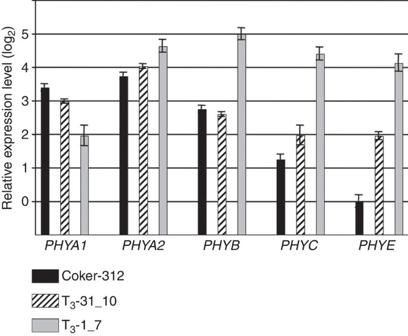Figure 6: Quantitative analysis of transcript abundance using phytochrome subfamily-specific qRT–PCR. The mean abundance ofPHYEin non-transformed Coker-312 was arbitrarily set at a value of 1. Relative expression of other transcripts is displayed on a log2scale. Error bars indicated the s.e.m. based on at least three biological replications. 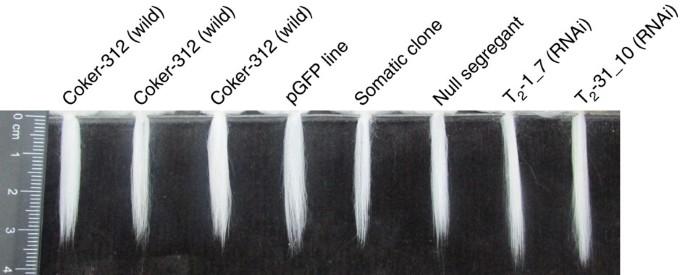The same plants were used for copy-number identification and relative expression analyses using qRT–PCR. Figure 5: Fibre staple length of control andPHYA1RNAi cotton plants. pGFP plant was transformed in our Uzbekistan laboratory with green fluorescent protein (GFP) construct (pBINmGFP5-ER ) used in cotton transformation12; somatically regenerated PCR-negative non-RNAi plant that escaped fromPHYA1RNAi vector transformation; pGFP, RNAi and somatic clones were regenerated from the same media, time and condition. Null segregant is non-RNAi plants segregated from T-1 and T-31 transformation events. Full size image Figure 5: Fibre staple length of control and PHYA1 RNAi cotton plants. pGFP plant was transformed in our Uzbekistan laboratory with green fluorescent protein (GFP) construct (pBINmGFP5-ER ) used in cotton transformation [12] ; somatically regenerated PCR-negative non-RNAi plant that escaped from PHYA1 RNAi vector transformation; pGFP, RNAi and somatic clones were regenerated from the same media, time and condition. Null segregant is non-RNAi plants segregated from T-1 and T-31 transformation events. Full size image Analysis of major fibre characteristics and cottonseed yield On the basis of phenotypic evaluation of T 2 -generation plants in the field in 2009, we selected two elite plant families, designated T 2 -1 and T 2 -31, for further characterization. These two independent RNAi transformants had directionally similar but quantitatively different phenotypic characteristics for traits such as boll maturation and hypocotyl length ( Supplementary Tables 1 and 3 ), root development ( Fig. 4c, d ) and some of the fibre quality traits, for example, microniare ( Table 1 ). Table 1 Fibre quality seed and yield traits averaged from 2009 and 2010 growing environments. Full size table In combined ANOVA ( Supplementary Table 4 ) of the 2009 and 2010 small replicated plot field evaluations, both of the RNAi families showed significantly increased (5%; ANOVA, P ≤0.01) upper half mean (UHM) fibre length ( Table 1 ; Figs 4a and 5 ), and improved MIC (4–8%; MIC, representing the thickness of cotton fibre), with no decrease in fibre uniformity, in comparisons with sibling plants lacking the RNAi construct (that is, null segregants) as well as non-transformed Coker-312. The modestly improved fibre strength (STR; 5%) and fibre elongation (ELO; the elasticity (%) of matured fibre) traits (2–10%) in RNAi families were statistically different (ANOVA, P ≤0.01) from non-transformed Coker-312, but not the null segregant control, suggesting possible effects of somaclonal variation and/or environmental interactions on these traits. However, trait differences between non-transformed Coker-312 and null segregant controls were not statistically significant at P ≤0.01 (ANOVA) in any of the traits tested, indicating that any effects of somaclonal variation or environmental differences were minor. MIC, ELO and fibre colour (+B) traits statistically differed (ANOVA, P ≤0.01) between T-1 and T-31 RNAi families. Genotype by environment interactions for major fibre quality traits evaluated in the two subsequent seasons were not significant at P ≤0.01 in combined ANOVA except for ELO (ANOVA, P =0.0006) and fibre colour (+B; ANOVA, P =0.0001) traits ( Supplementary Table 4 ). Selected T 2:3 RNAi families, examined over two seasons, showed small but statistically significant (ANOVA, P ≤0.01) decreases of up to 3% in lint percentage and up to a 10–12% decrease in lint index. However, the average number of fibres per seed ( Table 1 ) was not significantly decreased in PHYA1 RNAi lines (~10,492, ~10,289) when compared with the Coker-312 wild-type (~10,848) or the null segregant controls (~10,485). Overall, a statistically significant 3% increase in seed weight was observed in RNAi plants. The average seed cotton weight per boll significantly increased in RNAi genotypes (~6.37–6.41 g) compared with wild-type (~5.67 g) and null segregant (5.57 g) controls ( Table 1 ). Comparative measurements of the raw seed cotton weight per unit area from small replicated plots of T 3 and T 4 generations of elite RNAi families in the two subsequent seasons showed an average 10% yield increase over non-RNAi control plants ( Supplementary Table 5 ). Copy number of integrated RNAi vectors Vector-specific PCR amplification (see Supplementary Table 6 for primers) confirmed the insertion of the pHellsgate-8:: PHYA1 RNAi construct into the genomes of the selected T 3 RNAi lines ( Fig. 4b ). Quantitative PCR (qPCR) results based on standard curve ( Supplementary Table 7 ) showed that T 3 -1_7 plant have three copies while T 3 -31_10 plant contained two copies of pHellsgate-8:: PHYA1 RNAi construct in their genomes. As an additional control, we included genomic DNA from Bt-cotton that has a known single copy of the cry I transgene inserted in its genome ( Supplementary Table 8 ). Relative expression of cotton phytochrome genes Abundance of phytochrome transcripts in leaf tissues of non-transformed Coker-312 was highest in the PHYA subfamily ( PHYA2 > PHYA1 ), incrementally lower in PHYB and PHYC and lowest in PHYE ( Fig. 6 ; Supplementary Tables 9–11 ). In somatically regenerated transformants carrying the pHellsgate-8:: PHYA1 RNAi vector, PHYA1 transcript was suppressed by ~70% in T 3 -1_7 and ~25% in T 3 -31_10. The RNAi construct did not appear to suppress the expression of PHYA2 or other phytochrome genes, with the possible exception of a slight (~10%) downregulation of PHYB in T 3 -31_10. Unexpectedly, we detected 2- to 20-fold overexpression of PHYA2 , PHYB (in T 3 -1_7), PHYC and PHYE genes in both RNAi lines. The overexpression of the non-target phytochrome genes was more evident in the T 3 -1_7 line where the deeper suppression of PHYA1 gene expression was observed compared with T 3 -31_10. Figure 6: Quantitative analysis of transcript abundance using phytochrome subfamily-specific qRT–PCR. The mean abundance of PHYE in non-transformed Coker-312 was arbitrarily set at a value of 1. Relative expression of other transcripts is displayed on a log 2 scale. Error bars indicated the s.e.m. based on at least three biological replications. Full size image Except for ELO, Pearson’s R statistics between fibre traits described in Table 1 and relative quantity of cotton phytochrome transcripts ( Fig. 6 ; Supplementary Table 11 ) revealed negative (−0.6 to −1) or positive (0.54–0.98) correlations. For instance, a Pearson correlation between UHM and PHYA1 expression was equal to −0.854, UHM and PHYA2 was 0.859, UHM and PHYB was 0.611, UHM and PHYC was 0.68, and UHM and PHYE was 0.753. Transferability of phytochrome-specific RNAi effects We crossed T 0 -generation PHYA1 RNAi Coker-312 plants (including T-1 and T-31 RNAi families described herein) with several popular Upland cotton cultivars that are grown commercially in Uzbekistan. The F 1 and F 2 generation hybrids from these crosses (for example, sexual hybrids between AN-Boyovut-2 and T-1_7) had more vigorous vegetative growth ( Fig. 3b ), elongated petioles, elongated boll peduncles, elongated fruiting branches, more flowers and bolls, earlier flowering (5–10 days) and earlier boll maturity, and senescence-associated anthocyanin pigmentation in leaves and stems compared with the non-RNAi commercial control cultivars and null hybrid (Uzbek cultivar crossed with Coker-312) grown side by side in the same plots ( Supplementary Figs 7 and 8 ). In the F 2 and F 3 generation hybrids, major fibre quality traits were significantly improved, compared with the original cultivated variety and the null hybrid ( Fig. 3c ; Supplementary Fig. 9 ; Supplementary Table 12 ). For example, in the PHYA1 RNAi hybrid AN-Boyvut-2 × Coker-312_ T 0 -1, UHM was 1.29 inch, MIC was 4.36 and STR was 31.75 g/tex. These values were statistically different (ANOVA, P ≤0.05) from the original variety AN-Boyvut-2 and null hybrid (1.19 inch for UHM, greater than ~4.64 for MIC and less than 30.61 g/tex for STR, based on averages of two seasons of field evaluations). Similar trends in fibre trait improvement, as well as vigorous flowering and root development, were observed in F 2 and F 3 generations of crosses to several other Uzbek commercial cotton varieties ( Supplementary Fig. 10 ). The lint percentage (33.82%) and average number of fibres per seed (~12,661) were significantly decreased (ANOVA, P ≤0.05) in the RNAi × commercial variety hybrids compared with the null hybrid (34.04 lint% and ~12,979 fibres per seed), and the original cultivar (35.97 lint% and ~13,351 fibres per seed; Supplementary Table 12 ). However, the average seed cotton weight per boll was increased in RNAi hybrids (~6.58 g) compared with the non-hybrid cultivar (~6.08 g) and null hybrid (~6.13 g) controls ( Supplementary Table 12 ). We observed an average 17% increase in seed cotton yield ( Supplementary Table 5 ) per unit area over original non-RNAi variety, as can be clearly seen in the RNAi hybrid versus control plant rows shown in Supplementary Figs 7–10 . Phytochrome genes play key regulatory roles in a wide range of plant developmental processes [1] , [2] , [3] . As such, the manipulation of phytochrome gene function has long been considered as a promising avenue for the modification of economically important traits in crops [13] , [14] . For example, overexpression of a transgenic PHYA gene in tobacco resulted in suppression of shade avoidance and greater allocation to leaf growth, resulting in an improved leaf harvest index [15] . Overexpression of the Arabidopsis PHYB gene in transgenic potato ( Solanum tuberosum ) resulted in increased tuber yields [16] . Previously, we observed a statistical association (Logarithm of odds (LOD)=4.13; the Kruskal–Wallis test, P =0.0001) between a PHYA1 single nucleotide polymorphism marker and fibre quality in an interspecific cross between Pima S-7 (G. barbadens e) and Tamcot SP37 (G. hirsut um) consisting of 96 F 2 individuals [9] . We selected a unique PHYA1 -specific fragment for the RNAi construct based on our previous sequencing of the phytochrome gene family in cotton [10] . The 213 bp PHYA1 fragment used in this construct shared 87% nucleotide similarity with the cotton PHYA2 genes, 75% nucleotide similarity with Arabidopsis PHYA and only 50–59% nucleotide similarity with cotton PHYB, PHYC and PHYE genes. Since effective RNAi suppression typically requires 80–100% nucleotide identity [17] , we anticipated that our construct would only target the PHYA1 genes and perhaps PHYA 2 genes as well. Our results demonstrated that the suppression level of PHYA1 modified the expression of other phytochrome genes. Cross-regulation among the phytochrome genes has been observed in Arabidopsis and other plants. For example, Arabidopsis loss-of-function phyB mutants show reduced expression of PHYC in dark-grown tissues, and reduced PHYC , PHYD and PHYE in light-grown tissues [18] . In light-grown tissues from a sorghum phyB mutant, PHYA expression was increased in all light conditions tested [19] . These cross-regulatory effects may be the manifestations of a compensatory regulatory network [20] , [21] , [22] . In cotton, we observed a substantial increase in PHYB transcript in the strongest of our T 3 -1_7 RNAi line ( Fig. 6 ). This sharply contrasts with findings from Arabidopsis in which loss-of-function phyA mutations showed no increase in PHYB expression [23] . Similarly, both of the PHYA1 RNAi lines showed increased transcript levels for PHYA2 , PHYC and PHYE . These observations also contrast with Arabidopsis [18] , [23] , and indicate that the phytochrome regulatory network of cotton may have a fundamentally different dynamic architecture than that of Arabidopsis. While earlier observations suggested an effect of increased FR/R light ratio on fibre length and diameter [4] , and identified a preliminary association of PHYA1 with a fibre length QTL in cotton [9] , our results provide solid evidence of a molecular role for phytochromes in regulating cotton fibre traits. As cotton lacks the sophisticated molecular and genomic ‘tool kit’ of the model plant Arabidopsis, including facile Agrobacterium transformation [24] and comprehensive collections of knockout mutants [25] , it is not possible at this point to ascribe the fibre phenotypes directly to the suppression of PHYA1 or, alternatively, to the indirect effects of the increased levels of PHYA2 , PHYC and PHYE . In either case, enhancement of fibre length could occur because of a change in phytochrome-mediated plant hormone signalling [1] , [26] , [27] . Auxin (indole-3-acetic acid, IAA), abscisic acid, gibberellic acid, brassinosteroids, ethylene and cytokinin are known factors associated with fibre development [6] . For instance, recent spatiotemporal manipulation of auxin biosynthesis in developing cotton ovules showed enhancement of fibre yield and quality parameters [6] . There is well-supported evidence of molecular crosstalk between auxin and light signalling. Interactions of auxin with PHYA through phytochrome-dependent phosphorylation of auxin-related proteins, increases in auxin biosynthesis or regulation of auxin distribution [26] could explain the fibre length improvement in our PHYA RNAi plants [6] . Further, we previously observed that photomorphogenesis-related factors (for example, PHYC , SPA1 , FAR1 , COP1 , COP9 , CIP7 , CIP8 and RTP2 ) were targeted by putative ovule-derived short interfering RNAs during the initiation and elongation phases of fibre development [28] , thus indirectly supporting a role for light signalling in fibre traits. Our data suggested that some fibre traits (for example, ELO and STR) might be minimally affected by somaclonal variation. However, the major phenotypic variations (for example, fibre length, flowering, plant architecture, shoot and root developments, maturity and so on; Figs 1 , 2 , 3 , 4 , 5 ) observed among plants from different transformation events were correlated with the level of PHYA1 RNAi suppression, which could in turn be due to differences in RNAi copy number ( Supplementary Table 8 ), the positions of genome insertions or the arrangement of the transgene locus in the cotton genome. In our study, the T 3 -1_7 line had the most dramatic phenotypic effects, and also had the greater suppression of PHYA1 gene and the higher estimated copy number of the RNAi construct. Somaclonal variation resulting from extended tissue culture may have also contributed to the decreased lint percentage and lint index, as well as a non-significant decrease in the average number of fibres per seed in RNAi genotypes and in the null segregant. Further lint percentage decreases in RNAi plants might be directly associated with the average number of fibres per seed, or it could be influenced by the increased fineness of RNAi plant fibres. Improvements in fibre quality characteristics such as microniare, STR, uniformity index and others could also be the result of modified flowering time that made the plants better adapted to local environmental conditions. We also speculate that an early senescence of vegetative organs (in particular leaves) in the RNAi cotton lines may lead to an earlier mobilization of leaf cell nutrient resources, and transfer to the developing fruits, fostering simultaneous maturation of all cotton plant bolls, thus improving fibre quality. Moreover, increased yield may be due to some combination of more vigorous shoot growth (including greater numbers of fruiting branches, flowers and bolls, as well as improved seed cotton weight per boll) and root development (potentially improving water and nutrient assimilation) in RNAi plants. The multiple-fold overexpression of cotton PHYE (as well as PHYB in line T 3 -1_7) in PHYA1 RNAi plants might result in increased yield potential, as has been seen in tobacco [15] and potato [16] since PHYE is most closely related to PHYB , both functionally and phylogenetically [1] , [2] , [3] . This hypothesis is supported by the observation that both the potato PHYB -overexpressing lines [16] and our cotton PHYA1 RNAi suppression lines showed markedly increased anthocyanin production, particularly close to the time of senescence. The increased yield could also be associated with enhanced root development of RNAi lines, thus mediating better assimilation of soil nutrients or water. Early maturity and flowering of cotton also minimizes late season risks of insects/pathogen attacks and aids in proper timing of crop rotation (for example, wheat-cotton-wheat), potentially increasing farm incomes by reducing the input costs for fertilizers, water, insecticides and pesticides [29] . In particular, unfavourable late season weather conditions significantly decrease fibre quality parameters [29] . Early maturity of cotton cultivars is especially vital for cotton-growing plantations of northern latitudes with short cotton seasons such as Uzbekistan—the northernmost cotton growing country. Through manipulation of PHYA1 expression using RNAi, we have achieved simultaneous improvement of several important traits, such as fibre length and early maturity, without negatively affecting other key parameters such as yield—a goal that has largely eluded conventional breeding. For instance, introgression of superior fibre quality traits from Pima cotton ( G. barbadense ) into Upland ( G. hirsutum ) cultivars using interspecies genetic hybridization is challenging owing to segregation distortion and linkage drag that often results in introgressed progenies that are late maturing or have poor agronomic quality [30] . Application of RNAi has allowed us to effectively solve these fundamental problems, and rapidly improve maturity, flowering, yield and major fibre quality traits, thus transforming commercial Upland varieties into more long-stapled, productive and early-maturing cultivars. Coker-312 is the only G. hirsutum line that is easily amenable to tissue culture regeneration [12] , [31] , [32] ; however, it is not a commercially competitive fibre producer. While our RNAi construct was initially introduced and tested in Coker-312, a critical challenge was to show genetic stability and transferability of this construct and its resulting suite of traits to elite commercial cultivars. Using conventional sexual crosses, we successfully transferred the RNAi into the elite Uzbek commercial line AN-Boyovut-2 (which is well adapted for local growing conditions and cultivation practices). We succeeded in the efficient and stable transfer of the RNAi effects that were observed in original RNAi Coker-312 line, while maintaining the adaptive characteristics of the original cultivar, AN-Boyovut-2, thus developing a new superior cotton cultivar. While some small effects on fibre traits (for example, STR) may have been influenced by factors such as hybrid vigour (heterosis), environmental conditions and varietal background ( Supplementary Table 12 ), the dramatic improvements observed in RNAi hybrids (for example, UHM, MIC and STR) were not seen in variety × Coker-312 null-hybrid plants (that is, without the RNAi construct), and are therefore probably due to action of the RNAi transgene itself. Similar trend of key agronomic and fibre quality trait improvements in several other Uzbek Upland cultivar backgrounds ( Supplementary Fig. 10 ) further demonstrated the usefulness of PHYA1 RNAi for conventional cotton breeding. With the intent of future commercialization, later generations (F 4:5 ) of RNAi families with improved traits are being tested in larger field plots in Uzbekistan in 2012–2015. Thus, modification of cotton through modulation of phytochrome photoreceptor activity using RNAi not only provides a solution to a longstanding problem for conventional cotton breeders (fibre quality versus yield and early maturity), but may also lead to significantly increased income for cotton producers worldwide, thus opening a new paradigm in Upland cotton improvement. The demands for longer, finer and stronger cotton lint fibre, as well as early maturity, early flowering and improved seed cotton yield potential are key economic incentives in the global cotton market, and highlight the importance of our findings. Plant materials Plant materials used in this study were the somatically regenerable cotton genotype G. hirsutum line Coker-312 and its transgenic derivative lines, transformed with pHellsgate-8:: PHYA1 vector. To verify the transferability of the observed RNAi effects, we used several commercially important Uzbek cotton cultivars, for example, G. hirsutum cv. AN-Boyovut-2, C-6524, Namangan-77 and/or Toshkent-6 for the conventional genetic hybridization experiments with RNAi Coker-312 plants. RNAi vector construction For RNAi vector construction, cotton PHYA1 gene-specific primers with the attB sites (Gos_PHYA1attB1-F and Gos_PHYA1attB2-R) were designed ( Supplementary Table 6 ) and purchased from Integrated DNA Technologies Inc., (IA, USA). The specific cotton PHYA1 fragment (213 bp) was amplified from G. hirsutum (cv. TM-1) genomic DNA with KODHiFi high fidelity proofreading DNA polymerase (Novagen, USA) using non-attB gene-specific primers (PHYA1-F: 5′-GTGCTCGGAGTTAGTCCCATCAC-3′; PHYA1-R: 5′- GTCCGTATGATTGTTGATTGTCG-3′). The PCR was conducted according to the manufacturer’s instructions and protocol. The first round gene-specific PCR product sizes were verified using agarose gel electrophoresis; then, attB1 and attB2 sites were attached to the PCR products in a second round of PCR with attB-flanked gene-specific primers ( Supplementary Table 6 ). PCR products were purified with polyethylene glycol solution (containing 26% polyethylene glycol 8,000, 6.5 mM MgCl 2 and 0.6 mM sodium acetate pH 5.2) to remove remaining attB primers. Site-specific recombination between attB site-flanked gene fragment and the vector pDONOR221 (Invitrogen, USA) was conducted as described by Helliwell et al. [11] in a total reaction volume of 10 μl, with 2 μl BP clonase buffer (Invitrogen), 2 μl attB site-flanked PCR product, 150 ng plasmid vector and 2 μl BP clonase (Invitrogen). The reaction mix was incubated at 25 °C overnight and 2 μl of this recombination mix was transformed into chemically competent DH5-alpha Escherichia coli cells (Invitrogen). Transformed cells were grown in lysogeny broth (LB) agar plates containing 50 mg l −1 spectinomycin and colonies were subjected to plasmid isolation by the NaOH/SDS lysis method [33] and analysis by the PCR of the insertion with vector-specific M13 primers. Recombinations reaction between the pDONOR221-attB- PHYA1 and the pHellsgate-8 vector with 35S promoter [11] were conducted in a total volume of 10 μl, with 2 μl LR clonase buffer (Invitrogen), 2 μl recombinant pDONOR221-attB- PHYA1 (150 ng), 300 ng pHellsgate-8 and 2 μl LR clonase (Invitrogen). Reactions were incubated for overnight at room temperature, treated with proteinase K and a 2-μl aliquot was transformed into DH5-cells (Invitrogen). Cells were grown in LB plate containing selective antibiotic (spectinomycin) and colonies picked for verification of correct recombination with att B sites by restriction analyses with XhoI (for sense orientation site) and Xba (anti-sense orientation site). Positive clones were selected for further RNAi vector preparation as described by Helliwell et al. [11] RNAi vectors were transformed into Agrobacterium tumefaciens strain LBA4404 for plant transformation experiments. Cotton transformation and somatic embryogenesis We used a combination of available methodologies for cotton tissue culture [12] , [31] , [32] . Hypocotyl sections (5–7 mm thickness) from 1-week-old seedlings of Coker-312 were wounded with a laboratory razor and placed on P1 medium (4.31 g l −1 Murashige and Skoog basal salt mixture (MS salt), 0.4 mg l −1 thiamine HCl, 100 mg l −1 myoinositol, 0.75 mg l −1 MgCl 2 , 3% glucose, 0.2% phytagel, 5 mg l −1 N 6 -(2-isopentenyl) adenine, 0.1 mg l −1 1-naphthaleneacetic acid, pH 5.8). On the top of these wounded hypocotyl sections, 5 μl of a suspension of A. tumefaciens LBA4404 bearing the pHellsgate-8:: PHYA1 RNAi vector was applied, followed by an incubation at 22 °C for 72 h in the dark. The LBA4404 suspension bearing pHellsgate-8:: PHYA1 RNAi vector was grown in YEP medium (10 g l −1 Bacto peptone, 5 g l −1 NaCl, 10 g l −1 Bacto yeast extract, pH 7.0) containing rifampicin (10 m l −1 ) and spectinomycin (50 mg l −1 ) antibiotics. Bacterial cultures were grown in culture tubes for 36 h at 26 °C with shaking at 200 r.p.m. Cells from five tubes were pooled, harvested by centrifugation at 3,200 g for 10 min (Eppendorf 5810R, Germany) and resuspended in 10 ml of pre-induction medium (10 g l −1 glucose, 14.62 g l −1 2-(N-morpholino)ethanesulfonic acid, 20 ml l −1 sodium phosphate buffer pH 5.6 and 50 ml l −1 20 × AB salt stock [34] containing 100 μM acetosyringone). For controls, 5 μl sterile water was applied instead of bacterial suspension. After 72 h, infected and control hypocotyl sections were transferred to fresh P1 medium, containing kanamycin (50 mg l −1 ) and cephabol (500 mg l −1 ; analogue of clavamox), and cultures were grown under a 16-h photoperiod (10 μmol m −2 s −1 ). After 3 weeks, 3 mm callus tissues were transferred into new P7 medium (4.31 g l −1 MS salts, 0.4 mg l −1 thiamine HCL, 100 mg l −1 myoinositol, 0.75 mg l −1 MgCl 2 , 3% glucose, 0.2% phytagel, 0.1 mg l −1 (2-isopentenyl) adenine, and 5 mg l −1 1-naphthaleneacetic acid, pH 5.8) and sub-cultured onto fresh media monthly. Callus tissues less than 3 mm were kept in P1 medium for another 3 weeks and subsequently transferred to the P7 medium. After 16 weeks, to induce the somatic embryogenesis callus tissues grown on selective P7 medium were transferred to new modified medium R5 (4.31 g l −1 MS salt, 1 ml l −1 vitamins Gamborg solution, 1.9 g l −1 KNO 3, 0.75 mg l −1 MgCl 2 , 3% maltose and 0.2% phytagel) in which somatic embryos arose after 12–16 weeks. Somatic embryos 6–7 mm in size were transferred into modified SH1 (10 ml l −1 100 × micronutrients, 50 ml l −1 50 × macronutrients, 1 ml l −1 vitamin B5, 5 g l −1 sucrose, 15 g l −1 bactoagar and 2 g l −1 phytagel) medium and incubated in the dark for 10 days. After dehydration [32] and root initiation, embryos were transferred to new SH-2 medium (10 ml l −1 100 × micronutrients, 50 ml l −1 50 × macronutrients, 1 ml l −1 vitamin B5, 20 g l −1 sucrose, 1 g l −1 phytagel and 5 g l −1 agar) and grown for 10 days under a 16-h photoperiod (10 μmol m −2 s −1 ). After the development of initial roots and leaves, embryo plantlets were transferred to SH-3 medium (10 ml l −1 100 × micronutrients, 50 ml l −1 50 × macronutrients, 1 ml l −1 vitamin B5, 20 g l −1 sucrose, 1 g l −1 phytagel and 2.25 g l −1 agar) and grown with increased light (70 μmol m −2 s −1 ) for full development of roots and leaves. After 10 days, fully developed embryo plantlets were transferred into plastic containers with SH-3 medium and grown until the development of four to five leaves and additional roots. All reagents for cotton tissue culture were purchased from Phytotechnology Laboratories, USA. Identification of transformed plants using PCR Genomic DNAs were isolated from frozen leaf tissues using the method of Dellaporta et al. [35] Amplification reactions were performed in 50 μl volumes containing 4.5 μl 10 × PCR buffer with 1.5 mM MgCl 2 , 1 μl BSA, 0.5 μl 25 mM of a dATP, dGTP, dTTP and dCTP mix, 2.5 μl 50 ng ml −1 of each RNAi vector-specific 35S-F/PDK-R or PDK-F/OST-R primers pairs ( Supplementary Table 6 ), 1 μl 50 ng ml −1 template DNA and 0.5 U Taq DNA polymerase (Sigma, USA). Amplifications were carried out with an initial denaturation at 94 °C for 3 min followed by 45 cycles of 94 °C for 1 min, 55 °C for 1 min and 72 °C for 2 min. A final 5 min extension at 72 °C was then performed. For determining PCR product sizes, 2% agarose (Sigma) gel electrophoresis was carried out in 0.5 × TBE buffer. Gels were stained with ethidium bromide. RNAi plant evaluations and statistical analyses PCR-positive transformants and control plants were transferred to soil and grown in the greenhouse environment to produce self-pollinated T 1 seeds. PCR-positive PHYA1 RNAi embryonic plants were sexually hybridized with several popular Uzbekistan Upland cotton cultivars and F 1 hybrid plant seeds were harvested. Subsequently, 15–20 T 1 or F 1 seeds were germinated in small paper-soil pots in the greenhouse environment, and plants were checked to verify the presence of the transgene using PCR with RNAi vector-specific primers. PCR-positive T 1 and F 1 plants were transferred into larger pots and evaluated for flowering time, boll maturation and fibre staple length characteristics compared with non-transgenic Coker-312 plants grown in the same greenhouse environment. Flowering characteristics were determined from flowering time (the first flower opening date from planting) and number of opened flowers. Maturity was determined based on number of opened bolls (above 50%) per plant at the time of harvesting the bolls. Fibre length was measured manually in comparison with control Coker-312 genotype fibres or original non-RNAi Uzbek cultivar. Further, 40–45 T 2 or F 2 plants, derived from each superior quality T 1 or F 1 plant (single seed decent) of different transformation events, were grown as a family along side of 25 non-transgenic control Coker-312 plants in standard replicated field plot design in a two-row (60 × 30 cm 2 row-spacing) layout. Evaluations were conducted at the controlled field station (with no access of cross-pollinating insects) of the Institute of Genetics and Plant Experimental Biology, Tashkent, Uzbekistan in 2009. Plots were 6.3 × 1.2 m 2 . The average indices for hypocotyl length, number of opened flowers and opened bolls of each field-grown T 2 or F 2 RNAi family and control plants were recorded. First, flowers opened were tagged with date. All plants were self-pollinated to produce pure T 3 or F 3 generation seeds (by wrapping the petals with cotton threads before floral opening). In 2010, self-pollinated T 3 or F 3 generation seeds from two superior RNAi families (T 2 -1_7 and T 2 -31_10) and control plants were grown in the field station, Tashkent, Uzbekistan, with each family in 10 rows, 10 m long and 9 m wide plot, with 90 × 20 cm 2 row-spacing layout. Evaluations were performed with at least three replications for RNAi, RNAi hybrid and control plants. We measured yield potential by weighing the raw seed cotton yield from T 3 or F 3 RNAi cotton families and controls grown in the same field and environmental conditions. Lint percentage, the weight of 100 seeds (seed index) and lint index were measured manually from randomly chosen individual plants of each selected T 2:3 or F 2:3 RNAi family and control plants, taking seed cottons from the six fully matured bolls per plant. Root length of RNAi and control plants was measured 25 days after seed germination. Plastic pots were cut and roots were carefully washed. In addition, randomly chosen individual T 2:3 or F 2:3 plants from the field were dug at the flowering and boll maturation stages, roots were washed and root lengths were compared with control plants. Germination rates and hypocotyl lengths of T 2:4 generation RNAi plants and controls were measured in triplicate under light (16 h photoperiod, 100 μmol m −2 s −1 ) and dark conditions in the laboratory. Fibres of the second- and third-generation plants from replicated plots were ginned in small laboratory roller gin, and the main fibre quality traits of the same field-grown RNAi and control plants from 2009 and 2010, including UHM, MIC, STR, ELO, fibre uniformity, Rd and +B were measured using high volume instrumentation at the fibre-testing Centre ‘SIFAT’, Tashkent Uzbekistan and STRAR LAB at Knoxville, TN, USA. The number of fibres per seed was determined according to the methodology by Zhang et al. [36] in a triplicate experiment, averaged from the independently repeated counting performed by three different individuals using microscopy. The statistical significance of trait differences between RNAi families and control plants were tested in combined ANOVA using main effects and two-way interactions of Visual Statistics software (ViSta [37] ). Copy-number identification for the integrated RNAi sequence We followed the real-time qPCR (qRT–PCR) methodology [38] and calculations [39] to estimate the copy number of the PHYA1 RNAi vector integrated into the transformed cotton genomes. We cloned the GhUBC1 fragment into the plasmid vector pCR4 TOPO-TA following the manufacturer’s protocol and instructions (Invitrogen), which contains nptII gene as a selectable marker. This way, we obtained a reference plasmid vector containing both nptII and GhUBC1 gene for constructing a standard curve based on absolute copies of the plasmid vector ( Supplementary Table 7 ). We made 10-fold serial dilutions of plasmid vector and amplified target genes using qRT–PCR primer pairs and probes ( Supplementary Table 6 ). qRT–PCR was carried out in an Applied Biosystems 7500 real-time PCR system (Applied Biosystems, Foster City, USA). PCR reactions were performed in a 12.5-μl volume with the following standard programme recommended by the manufacturer: 95 °C for 10 min, followed by 40 cycles of 95 °C for 15 s and 60 °C for 1 min. Each 12.5 μl reaction mixture contained 6.25 μl Master Mix (2 × ), 0.25 μl (200 nM) of each primer (10 μM), 1 μl (40 nM) of probe (0.5 μM), 4 μl of template DNA sample (0.2 pg–20 ng) and 0.75 μl sterile deionized water. A 2 × PCR Master Mix contained No AmpErase UNG, AmpliTaq Gold DNA polymerase, deoxynucleoside triphosphates with dUTP and Taq Man reaction buffer with magnesium chloride (Applied Biosystems). Average C t values were plotted against log of absolute copy numbers to obtain standard curves. Six replicates were conducted to construct standard curves for each target gene. Efficiencies of amplification were calculated based on slopes of standard curves with the following formula: E =10 (−1/slpoe) −1 (refs 38 , 40 ). The copy-number calculation was performed as described by Weng et al. [39] using the equation X 0 / R 0 =10 [( C t, X − IX )/ SX )]−[( C t, R − IR )/ SR ] , where X is nptII , R is UBC1 , I is intercept of the standard curve, S is slope of the standard curve for target ( X ) and reference ( R ) genes [39] . X 0 / R 0 values were used directly (that is, without doubling) for copy-number estimation since our samples were T 3 -generation plants, and not T 0 , as was the case in Weng et al. [39] Coefficient of variation in copy-number estimates was calculated from coefficient of variation estimates for GhUBC1 (endogenous control) and nptII (target gene). RNA isolation and quantitative real-time PCR Total RNAs were isolated from leaf tissues using combination of protocols described by Suzuki et al. [41] and Wu et al. [42] RNAs were isolated from the same control and RNAi plants that were used for copy-number identification and detailed phenotypic evaluations. Briefly, 100 mg of fresh leaf tissues was frozen in liquid N 2 and powdered using a pestle and mortar, followed by addition of 2 ml extraction buffer of Wu et al. [42] , heated to 80 °C and with 10 mM (1.54 mg ml −1 ) dithiothreitol freshly added. Then, 60 μl of 25 mg ml −1 proteinase K was added to the homogenate and ground further to mix. The homogenate was then transferred to 2 ml plastic tubes, incubated at room temperature for 15 min, and was then centrifuged (Eppendorf 5415R, Germany) at top speed for 20 min at 4 °C. The supernatant was transferred to fresh 2 ml tubes and RNA was isolated with a conventional water-saturated phenol:chloroform-isoamylacohol RNA precipitation procedure [41] , [43] . From this point, all steps were exactly as described and optimized by Suzuki et al. [41] The resulting RNA pellet was washed with 75% (v/v) ethanol, air-dried and dissolved in sterile diethylpyrocarbonate-treated water. The integrity of RNA was checked and judged by the presence and intensity of ribosomal RNA bands on a 1% agarose gel containing 2.2 M of formaldehyde in the presence of ethidium bromide [44] . RNA samples were treated with RNAase-free DNAase I (Ambion, USA) according to the manufacturer’s protocol and repurified with additional purification steps using acid phenol:chloroform (5:1; Ambion) and ethanol precipitation. The concentrations of total RNA samples were quantified using spectrophotometer (GENESYS 10UV, Thermo Scientific, USA). The first-strand complementary DNAs were synthesized from ~2 μg total RNAs using an Avian RT cDNA kit (Sigma) with random nonamer primers according to the manufacturer’s protocol. The first-strand cDNAs were diluted 1:15 with sterile water and used in expression analyses. RT–PCR reactions were carried out with intron-specific primer pairs [45] (A1341F/R; Supplementary Table S6 ) to check for DNA contamination, and with primers for catalytic subunit of protein phosphatase 2A gene of cotton ( GhPP2A1 ) [46] to check the quality of the cDNAs synthesized. RT–PCR reactions were carried out using an RT–PCR kit (Sigma) according to the manufacturer’s protocol. Samples were subjected to qRT–PCR only if they failed to amplify intronic primer pairs, but successfully amplified the endogenous ( GhPP2A1 ) reference gene. To identify RNAi influence in the expression of cotton phytochrome genes, we utilized a qRT–PCR method using SYBR green-based amplicon detection and primer pairs shown in Supplementary Table 6 . qRT–PCR was carried out in an Applied Biosystems 7500 real-time PCR system (Applied Biosystems). PCR reactions were performed in a 25-μl volume with the following cycling conditions: 95 °C for 10 min, followed by 40 cycles of 95 °C for 15 s and 65 °C for 45 s. Each 25 μl reaction mixture contained 12.5 μl SYBR Green Master Mix (2 × ), 0.35 μl (140 nM) of each primer (10 μM), 6 μl of template 1:15 times diluted cDNA template and 5.8 μl sterile deionized water. A 2 × SYBR Green PCR master mix contained No AmpErase UNG, AmpliTaq Gold DNA polymerase, deoxynucleoside triphosphates with dUTP and SYBR Green reaction buffer with magnesium chloride (Applied Biosystems). Post real-time PCR dissociation curves were constructed for each primer pairs and used to rule out primer-dimers, genomic DNA contamination and mis-annealing. Analysis of qRT–PCR amplifications was conducted using 7500 System SDS v1.4 Software (Applied Biosystems). For creation of standard curves for each gene used in qRT–PCR analysis, twofold dilution series (1 × , 2 × up to 128 × ) of 1:15 diluted cDNA from control Coker-312 was created. Average C t values from, at least, two replicates were plotted against log of starting amount to obtain standard curves. Efficiencies of amplification were calculated based on slopes of standard curves with the following formula: E =10 (−1/slope) −1 (refs 38 , 40 ). Slope and intercept indices from the standard curves obtained for each gene analysed were used to calculate log input amount (Log input amount=(Average C t target gene − Intercept target gene )/Slope target gene ); then, the input amount was calculated using 10 log input amount . Input amounts obtained for phytochrome genes were divided by the input amount of GhPP2A1 . The relative quantity of the target genes was then calculated by dividing the normalized quantity of target gene expression in RNAi plants by the normalized quantity of the same gene expression in a control plant, chosen as a calibrator. Coefficient of variation was calculated from coefficient of variation estimates for GhPP2A1 and each of the phytochromes. How to cite this article: Abdurakhmonov, I. Y. et al. Phytochrome RNAi enhances major fibre quality and agronomic traits of the cotton Gossypium hirsutum L. Nat. Commun. 5:3062 doi: 10.1038/ncomms4062 (2014).